Engineering near-infrared single-photon emitters with optically active spins in ultrapure silicon carbide Vacancy-related centres in silicon carbide are attracting growing attention because of their appealing optical and spin properties. These atomic-scale defects can be created using electron or neutron irradiation; however, their precise engineering has not been demonstrated yet. Here, silicon vacancies are generated in a nuclear reactor and their density is controlled over eight orders of magnitude within an accuracy down to a single vacancy level. An isolated silicon vacancy serves as a near-infrared photostable single-photon emitter, operating even at room temperature. The vacancy spins can be manipulated using an optically detected magnetic resonance technique, and we determine the transition rates and absorption cross-section, describing the intensity-dependent photophysics of these emitters. The on-demand engineering of optically active spins in technologically friendly materials is a crucial step toward implementation of both maser amplifiers, requiring high-density spin ensembles, and qubits based on single spins. Quantum emitters hosted in crystalline lattices are highly attractive candidates for quantum information processing [1] , secure networks [2] , [3] and nanosensing [4] , [5] . For many of these applications it is necessary to have control over single emitters with long spin coherence times. Such single quantum systems have been realized using quantum dots [6] , colour centres in diamond [7] , dopants in nanostructures [8] and molecules [9] . More recently, ensemble emitters with spin dephasing times in the order of microseconds and room-temperature optically detectable magnetic resonance (ODMR) have been identified in silicon carbide (SiC) [10] , [11] , [12] , a compound being highly compatible to up-to-date semiconductor device technology. Until recently, however, the engineering of such spin centres in SiC on the single-emitter level has remained elusive [13] . Silicon vacancy ( V Si )-related defects in SiC have some advantages compared with other solid-state single-photon emitters. In particular, the zero-phonon lines (ZPLs) of V Si -related defects in 4H and 6H polytypes of SiC present spectrally narrow features at near-infrared (NIR) wavelengths ( λ ZPL =850–1,200 nm) [10] , [14] , [15] , [16] . Rayleigh scattering losses in photonic structures are inversely proportional to the fourth power of the wavelength [17] , [18] , giving almost one order of magnitude lower losses for these defects compared with the nitrogen-vacancy defect in diamond ( λ ZPL =637 nm) [19] or the carbon antisite-vacancy pair in SiC ( λ ZPL =660 nm) [20] . Similarly, scattering losses at interfaces and signal attenuation in optical fibers decrease with wavelength as well. Furthermore, V Si -related defects in SiC can be integrated with existing optoelectronic devices [21] and, in contrast to GaAs-based quantum dots [22] , operate even at room temperature. Here, we demonstrate the control of spin centre density in ultrapure SiC over eight orders of magnitude, from below 10 9 to above 10 16 cm −3 using neutron irradiation. For a low irradiation fluence, a fully photostable, room temperature, NIR single-photon emitter can clearly be isolated, demonstrating no bleaching even after 10 14 excitation cycles. Based on their spectroscopic fingerprints, these centres are identified as silicon vacancies, which can potentially be used as qubits [16] , spin sensors [23] and maser amplifiers [12] . Confocal microscopy The 4H-SiC unit cell with a single V Si defect is shown in Fig. 1a . The dangling bonds of four C atoms with the absent Si atom result in formation of energy levels within the forbidden gap (3.23 eV) of 4H-SiC [24] , [25] . In case of negatively charged V Si , five electrons form a spin quadruplet ( S =3/2) in the ground state [12] , [26] . To excite these defects we use sub-band gap excitation of SiC at a laser wavelength of 785 nm ( hν =1.58 eV), which is close to their optimal excitation wavelength [27] . At room temperature, the V Si defects emit in the NIR spectral range from 800 to 1,100 nm. At cryogenic temperatures, two distinct ZPLs at λ ZPL =862 nm (V1) and λ ZPL =917 nm (V2), associated with two different crystallographic sites in 4H-SiC, are observed in the photoluminescence (PL) spectrum [28] , which can be used as spectroscopic fingerprints of V Si . 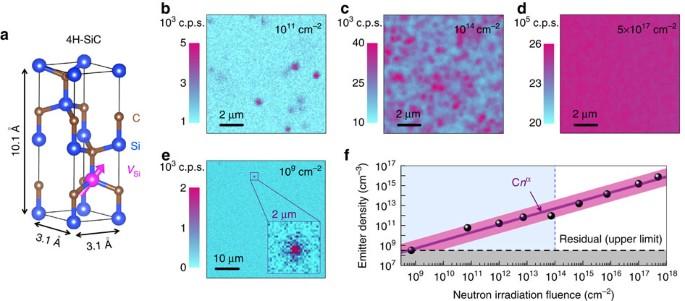Figure 1: Generation ofVSidefects in ultrapure 4H-SiC samples by neutron irradiation. (a) A scheme of the 4H-SiC unit cell with a singleVSidefect. (b–d) Confocal microscopy raster scans (10 × 10 μm2) for different neutron irradiation fluences: (b)n=1 × 1011cm−2, (c)n=1 × 1014cm−2and (d)n=5 × 1017cm−2. (e) A confocal microscopy raster scan (50 × 50 μm2) with a singleVSidefect (shown in the inset) forn=1 × 109cm−2. (f) Concentration of single-photon emittersas a function of the irradiation fluence. For low irradiation fluences up to the vertical dashed line, the concentration is found by direct count of emitters in the given volume. The solid line is a fit towithα=0.8. Figure 1: Generation of V Si defects in ultrapure 4H-SiC samples by neutron irradiation. ( a ) A scheme of the 4H-SiC unit cell with a single V Si defect. ( b – d ) Confocal microscopy raster scans (10 × 10 μm 2 ) for different neutron irradiation fluences: ( b ) n =1 × 10 11 cm −2 , ( c ) n =1 × 10 14 cm −2 and ( d ) n =5 × 10 17 cm −2 . ( e ) A confocal microscopy raster scan (50 × 50 μm 2 ) with a single V Si defect (shown in the inset) for n =1 × 10 9 cm −2 . ( f ) Concentration of single-photon emitters as a function of the irradiation fluence. For low irradiation fluences up to the vertical dashed line, the concentration is found by direct count of emitters in the given volume. The solid line is a fit to with α =0.8. Full size image To control the V Si density in a high-quality 110μm thick 4H-SiC epitaxial layer [27] , we used neutron irradiation (0.18 MeV< E n <2.5 MeV) in a fission reactor. The irradiation fluence was varied over more than eight orders of magnitude, from 10 9 to 5 × 10 17 cm −2 ( Fig. 1 ). Some parts of the generated V Si defects are negatively charged because of the presence of residual N donors (5.0 × 10 14 cm −3 ). Additionally, the neutron transmutation doping may play a role [29] , [30] . Such an unusual doping mechanism is caused by a nuclear reaction 30 Si(n, γ ) 31 Si→ 31 P+β − , when the capture of a neutron by the nuclear isotope 30 Si (natural abundance 3.2%) leads to the formation of an unstable isotope 31 Si. Followed by beta decay, it is converted into the stable isotope 31 P, resulting in additional n-type doping of SiC. A PL confocal raster scan (10 × 10 μm 2 ) on a sample irradiated with a low fluence of n =1 × 10 11 cm −2 is presented in Fig. 1b . The PL is detected in the spectral range from 875 nm (owing to a longpass (LP) filter) to 1,050 nm (limited by the sensitivity of Si avalanche photodiodes (APDs)). Four, nearly diffraction-limited spots (full-width at half-maximum of ∼ 500 nm) are clearly seen in this scan. With rising irradiation fluence to n =1 × 10 14 cm −2 the number of PL spots increases as well ( Fig. 1c ). For the highest irradiation fluence of n =5 × 10 17 cm −2 , single PL spots cannot be resolved anymore and the PL spatial distribution becomes highly homogeneous ( Fig. 1d ). Remarkably, in the negligibly weak irradiated sample (fluence of 1 × 10 9 cm −2 ) only one PL spot is found in the 50 × 50 μm 2 raster scan ( Fig. 1e ). The single spots are also restricted along the optical axis as shown in Fig. 2a . Below we unambiguously prove that these intensity spots are due to the emission from single V Si defects. 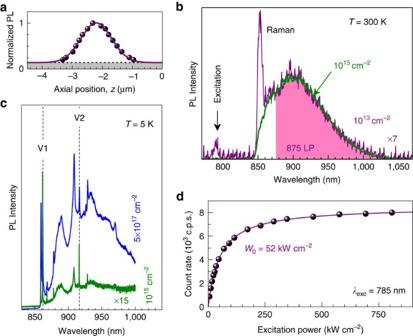Figure 2: NIR emission of a singleVSidefect in 4H-SiC. (a) PL line scan through a singleVSidefect. The top of the undoped 4H-SiC layer is placed atZ=0 μm. Integrated PL is obtained with a LP filter at 875 nm. The solid line is a Gauss fit with a full-width at half-maximum of 1.2 μm. (b) Room temperature PL spectrum of a singleVSidefect (n=1013cm−2) in comparison to aVSiensemble (n=1015cm−2). An 850 nm LP filter is used to suppress the excitation at 785 nm. An additional LP filter at 875 nm can be used to suppress a Raman line (LO phonon). (c) Low-temperature PL spectra ofVSidefects for different irradiation fluences. Two ZPLs, labeled as V1 and V2 (vertical dashed lines), are characteristic for two types of theVSidefect in 4H-SiC. (d) Photon count rate of a singleVSidefect as a function of excitation power density. The solid line is a fit to Equation (1) withW0=52 kW cm−2. Figure 2: NIR emission of a single V Si defect in 4H-SiC. ( a ) PL line scan through a single V Si defect. The top of the undoped 4H-SiC layer is placed at Z =0 μm. Integrated PL is obtained with a LP filter at 875 nm. The solid line is a Gauss fit with a full-width at half-maximum of 1.2 μm. ( b ) Room temperature PL spectrum of a single V Si defect ( n =10 13 cm −2 ) in comparison to a V Si ensemble ( n =10 15 cm −2 ). An 850 nm LP filter is used to suppress the excitation at 785 nm. An additional LP filter at 875 nm can be used to suppress a Raman line (LO phonon). ( c ) Low-temperature PL spectra of V Si defects for different irradiation fluences. Two ZPLs, labeled as V1 and V2 (vertical dashed lines), are characteristic for two types of the V Si defect in 4H-SiC. ( d ) Photon count rate of a single V Si defect as a function of excitation power density. The solid line is a fit to Equation (1) with W 0 =52 kW cm −2 . Full size image Defect density In order to find the density of single V Si photon emitters the following procedure is used. Up to the irradiation fluence of n =1 × 10 14 cm −2 we directly count the number of PL spots in the detection volume, given by the scanned area and the focus depth, the latter is about 1.2 μm according to Fig. 2a . For this irradiation fluence we also measure the integrated PL intensity collected from an area of ∼ 100 μm 2 . This PL is used as a reference to calculate the emitter density in the strongly irradiated samples by comparing their PL intensities. The results are presented in Fig. 1f . For the lowest irradiation fluence the defect density is , which can be taken as the upper limit of residual V Si concentration in our 4H-SiC sample. The concentration after the highest irradiation fluence constitutes . The real value can be even higher due to the generation of other types of defects with nonradiative recombination channels leading to a reduction of the PL intensity. The irradiation fluence dependence follows quite well a power law with α =0.8±0.1, as shown by the solid line in Fig. 1f . This empirical power law can be used for the calculation of the required irradiation fluence to create silicon vacancy of desired concentration. Theoretical modeling of the defect creation process is beyond the scope of this paper. Qualitatively, the sublinear dependence can be explained by the creation of some other types of defects at the silicon sites of the SiC lattice, such that at these sites a silicon vacancy cannot be created. However, this effect is relatively weak as α is close to one. To identify the type of generated defects, we measure the PL spectra for different irradiation fluences. The spectrum from a single centre is identical to the ensemble emission ( Fig. 2b ). Here we use a LP filter 850 nm to suppress the excitation light at 785 nm in the detection path. The LO phonon Raman line of 4H-SiC at 850 nm is independent of the irradiation fluence and hence is masked by the stronger PL band for n =10 15 cm −2 . We therefore use an additional LP filter 875 nm when investigating single centres. The PL spectra recorded at low temperature ( T =5 K) are presented in Fig. 2c . Two characteristic lines at 861.4 and 916.3 nm are clearly visible for different irradiation fluences. These lines coincide with the V1 and V2 ZPLs [28] , proving that the PL originates from the V Si defects in 4H-SiC. These lines have different intensity, which may be due to their different polarization [14] as in our experiments we are sensitive to the dipoles, which are polarized perpendicular to the c axis of SiC. Single defect characterization As expected for single defect centres, the PL intensity I saturates with increasing excitation power density W ( Fig. 2d ). After subtracting the linear background contribution and APD dark counts, it follows: Here, W 0 =52 kW cm −2 is the saturation power density exposed to the sample, corresponding to the laser power P 0 =0.3 mW at the objective entrance aperture. The saturation PL intensity varies slightly from spot to spot and in Fig. 2d yields I max =8.5 × 10 3 counts per second (c.p.s.). As a next step, we perform the Hanbury Brown and Twiss interferometry experiment, that is, the time correlation measurement of photon detection by two APDs. This is a frequently used method to verify single-photon emission [19] , [20] . The second-order correlation functions g (2) ( τ ), recorded over several hours for different W , are shown in Fig. 3b (see also Supplementary Note 2 ). The most important feature is the dip at zero time delay ( τ =0). For the lowest excitation, we obtain g (2) (0)=0.23±0.07<0.5, which denotes clearly the nonclassical behavior of a single-photon emitter. In addition to the antibunching for | τ | < 15 ns, there is also bunching for | τ | > 15 ns. To explain such a behavior at least three levels have to be involved ( Fig. 3a ). 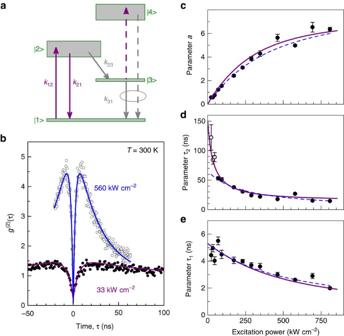Figure 3: Intensity correlation measurements at room temperature. (a) A four-level model of theVSidefect with radiative recombination from the excited state |2〉 to the ground state |1〉 and nonradiative relaxation through the metastable state |3〉, which in turn can be optically activated to another excited state |4〉. (b) Correlation functionsg(2)(τ) recorded at two different excitation power densitiesW<W0andW≫W0. The solid lines are fits to Equations (2) (c–e) Fit parametersa,τ1andτ2of the antibunching curve as a function of excitation power density. The dashed and solid lines are fits to three-level and four-level model respectively, as discussed in the text. Figure 3: Intensity correlation measurements at room temperature. ( a ) A four-level model of the V Si defect with radiative recombination from the excited state |2〉 to the ground state |1〉 and nonradiative relaxation through the metastable state |3〉, which in turn can be optically activated to another excited state |4〉. ( b ) Correlation functions g (2) ( τ ) recorded at two different excitation power densities W < W 0 and W ≫ W 0 . The solid lines are fits to Equations (2) ( c – e ) Fit parameters a , τ 1 and τ 2 of the antibunching curve as a function of excitation power density. The dashed and solid lines are fits to three-level and four-level model respectively, as discussed in the text. Full size image The second-order correlation function can be well described using as shown by the solid lines in Fig. 3b . The power dependencies of parameters a , τ 2 and τ 1 are presented in Fig. 3c–e , respectively. We use the same three-level model as for the colour centres in diamond [19] , [31] , [32] to fit these dependencies. This model describes reasonably well the bunching amplitude a ( W ) (the dashed line in Fig. 3c ) and the antibunching decay time τ 1 ( W ) (the dashed line in Fig. 3e ). The transition rates obtained using these fits are summarized in Table 1 . However, the relatively long bunching decay time τ 2 ( W ) for W <100 kW cm −2 is not well reproduced at low excitation powers within this model (the dashed line in Fig. 3d ). A possible explanation is that a deshelving process of the metastable state |3〉 may occur under optical excitation [32] . Table 1 Transition rates k ij and absorption cross-section σ governing the population dynamics of V Si . Full size table To describe the experimental data of Fig. 3 we consider a four-level model, where optical excitation from the metastable state to a higher-lying state and subsequent relaxation to the ground state occur ( Fig. 3a ). This results in intensity-dependent rate k 31 , saturating for high W following [32] We use the procedure described in the Methods section to find all the transition rates k ij and the results are summarized in Table 1 . Using this approach we achieve a very good agreement with our experimental data (the solid lines in Fig. 3c–e ). Remarkably, the excited state lifetime ( k 21 + k 23 ) −1 =5.3 ns agrees well with the PL decay time of 6.1 ns observed in time-resolved experiments [27] and is significantly longer than that of the band-to-band transition in semiconductor nanostructures [33] . Photostability is an important characteristic of a single-photon emitter. The PL time trace of a single V Si defect are shown in Fig. 4a . For a sampling bin to δt =100 ms, the count rate remains constant over minutes. To examine the photostability on a shorter time scale, the sampling bin is reduced to δt =1 ms. The number of detected photons per sampling bin is 10 in this case, and the time trace demonstrates statistical fluctuations without any indication of blinking ( Fig. 4b ). It should be indicated that blinking on much shorter time scales, if occurs, would not be detected in this case. We have also investigated a single V Si emitter over more than 1 week under continuous excitation and did not observe photobleaching. Assuming that the excitation occurs on average every 10 ns, this corresponds to 10 14 excitation cycles. 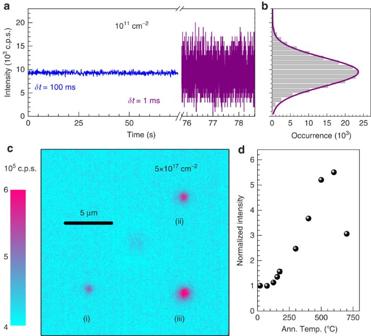Figure 4: Photostability ofVSidefects. (a) PL time traces with sampling binsδt=100 ms andδt=1ms, obtained on a singleVSidefect under excitation power density of 1,400 kW cm−2. (b) Corresponding count rate histogram forδt=1 ms. The solid line is a Gauss fit. (c) A confocal microscopy raster scan (20 × 20 μm2) recorded after laser illumination of different spots for 120 min: spot (i)P=0.5 mW; spot (ii)P=1.5 mW; and spot (iii)P=3.5 mW. (d) Relative change of theVSiPL intensity as a function of annealing temperature. TheVSidensity before annealing is. Figure 4: Photostability of V Si defects. ( a ) PL time traces with sampling bins δt =100 ms and δt =1ms, obtained on a single V Si defect under excitation power density of 1,400 kW cm −2 . ( b ) Corresponding count rate histogram for δt =1 ms. The solid line is a Gauss fit. ( c ) A confocal microscopy raster scan (20 × 20 μm 2 ) recorded after laser illumination of different spots for 120 min: spot (i) P =0.5 mW; spot (ii) P =1.5 mW; and spot (iii) P =3.5 mW. ( d ) Relative change of the V Si PL intensity as a function of annealing temperature. The V Si density before annealing is . Full size image The maximum count rate of a single V Si emitter in Fig. 4a is about 10 4 c.p.s. Using an optimized detection scheme with high detection efficiency of single photons as in the visible spectral range and with high optical transmission (above 90%) in the NIR, the count rate of about 4 × 10 4 c.p.s. should be achievable. However, this count rate is still lower as expected from the transition rates of Table 1 . This discrepancy can partially been explained by a relatively high refractive index of SiC ( n r =2.6), resulting in a large fraction of photons being restricted within the crystal due to the total internal reflection. To overcome this problem, one can either fabricate a solid immersion lens or use nanocrystals. In this case, together with optimized detection scheme a count rate above 10 5 c.p.s. is feasible. Laser annealing Finally we found that in the highly irradiated sample the PL intensity increases locally upon laser illumination. To demonstrate this effect, the laser light of different intensities was focused sequently on three different spots and remained there for 120 min, respectively. A confocal raster scan, performed at low laser power after such a procedure, demonstrates clearly a PL enhancement for each spot, as shown in Fig. 4c . For the highest laser power (spot (iii) in Fig. 4c ) this enhancement is ∼ 25%. There are two possible mechanisms of this effect. One of them is that the laser changes the charge state of the defects. Remarkably, the generated pattern of Fig. 4c remains over many hours, indicating that discharging in the dark should also occur on the same time scale. Alternatively, the focused laser beam can locally heat up the sample, resulting in atomic displacements and thus in disappearance or/and transformation of some other types of intrinsic defects (for instance, recombination of Frenkel pairs or migration of interstitials) [34] , generated upon neutron irradiation. These defects may serve as nonradiative recombination channels or as charge traps, switching off the V Si defects in close proximity. To show that heating indeed results in PL enhancement, we perform complementary annealing experiments by increasing stepwise the temperature and monitoring the integral PL intensity after each step. We prove that the PL spectrum remains unchanged ( Supplementary Fig. 2 ). The results are summarized in Fig. 4d , showing the overall PL enhancement by a factor of 5.5. This corresponds to and demonstrates that V Si defects can be created at high density in a controlled manner, as required, for instance, for the implementation of a SiC maser [12] . As has been mentioned in the introductory part, the generation of optically active spins is important for solid-state quantum computing and communications, sensing, precision measurement and so on [1] , [2] , [3] , [4] , [5] , [12] , [16] , [23] . Very recently, single emitters in the visible spectral range have been isolated in SiC wafers [20] and nanoparticles [35] . However, these emitters do not reveal such spin properties. To demonstrate that the V Si emitters engineered in the present work possess optically active spins, we perform ODMR experiments at room temperature ( Fig. 5 ). The ODMR maximum is observed at 71 MHz, corresponding well to the zero-field spin splitting of V Si (V2) in 4H-SiC in much dense V Si ensemble [23] . The experiment of Fig. 5 has been performed on the sample with irradiation fluence of 10 16 cm −2 , corresponding to ∼ 10 4 simultaneously detected V Si spins, as follows from Fig. 1f . This approach can be used to probe single spins as well, but with correspondingly increased readout time. 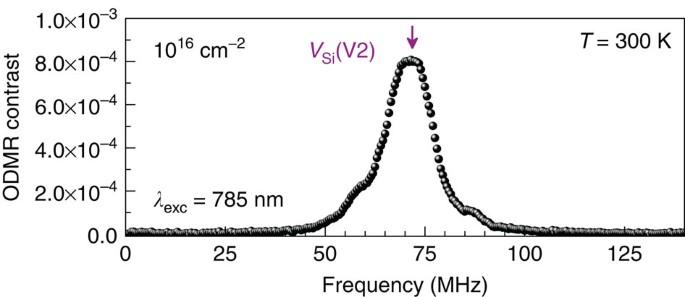Figure 5: Room-temperature ODMR spectrum of∼104VSidefects. The side peaks are due to uncompensated weak magnetic fields. Figure 5: Room-temperature ODMR spectrum of ∼ 10 4 V Si defects. The side peaks are due to uncompensated weak magnetic fields. Full size image In our experiments, we precisely control the concentration of V Si defects in ultrapure 4H-SiC down to single defect level. This approach can be used to deterministically incorporate [36] these atomic-scale defects in electronic [21] and photonic structures [37] as well as in nanocrystals [38] . Together with their extremely narrow optical resonances (on the order of 0.01 nm at low temperature [16] ) and recently demonstrated optically detected spin resonances at ambient conditions [23] , our results open exciting opportunities for various quantum applications with spin–photon interface. Note, when the manuscript was in the reviewing process, we learnt about two papers where the coherent control of single spins in SiC is reported [39] , [40] . Using a solid immersion lens, a count rate of 4 × 10 4 c.p.s. has been achieved [40] , supporting the conclusions drawn here. Samples The 4H-SiC sample has been purchased from CREE. A high purity (residual nitrogen doping below 5.0 × 10 14 cm −3 ) layer of 110 μm thickness was epitaxially grown on a 2-inch n-type 4H-SiC wafer. The layer is covered by a 5μm thick n-type 4H-SiC layer and a 2μm thick p-type 4H-SiC layer. The wafer was diced in 4 mm × 2 mm pieces, which were then irradiated in a TRIGA Mark-II nuclear reactor, with neutron energies in the range of 0.18 MeV< E n <2.5 MeV (see also Supplementary Note 1 ). Further information on the reactor is available at http://ati.tuwien.ac.at/reactor/EN/ . The sample with the highest neutron irradiation fluence of 5 × 10 17 cm −2 was thermally annealed in several steps from 125 to 700 °C for a time of 90 min, respectively. The heating was either performed on a heat stage (125–200 °C) or in an oven (300–700 °C). Experimental setup Samples were investigated with a home-build confocal microscope ( Supplementary Fig. 1 ) and a cw 785 nm laser was used for excitation. A three-dimensional piezo unit (nPoint) was used to move the SiC sample in lateral and axial directions. The excitation beam was focused onto the samples by a high aperture (NA=1.49) oil immersion microscope objective (UAPON 100XOTIRF, Olympus) with optical transmission in the NIR of about 60%. Collimated optical response of the sample was collected by the same objective and guided through a 30 or 75 μm pinhole (Thorlabs) followed by a 850 and 875 nm LP filter (Edmund Optics). Time correlated single-photon counting (TCSPC) was recorded by a Hanbury Brown and Twiss setup consisting of two APDs (Count-100C-FC, Laser-components GmbH) with a quantum efficiency of ∼ 0.3 at the signal wavelength and <100 c.p.s. in the dark and a 16-channel photon correlator card (DPC-230, Becker & Hickl GmbH) with a time resolution of at least 165 ps. The low-temperature PL spectra were measured at 5 K in a cryostat (MicrostatHe, Oxford Instruments) built into a confocal Raman spectrometer (LabRAM HR, Horiba). The excitation wavelength was 633 nm. In the ODMR experiment, the radio frequency radiation provided by a signal generator is amplified and guided to a thin copper wire terminated with a 50Ohm impedance. We use a standard lock-in detection scheme, described elsewhere [23] . Fitting procedure In order to find the transition rates k ij of the four-level model in Fig. 3a , we follow closely the approach applied to describe the photophysics of the silicon-vacancy colour centre in diamond [32] . First, we take the limiting values for W → 0 and W =800 kW cm −2 ≫ W 0 as an approximation for W →∞ and obtain τ 1 0 =5.3 ns, τ 2 0 =150 ns, τ 2 ∞ =14.5 ns and a ∞ =6.4. Under the assumption we calculate The excitation rate of V Si is proportional to the laser power density k 12 = σW , where the absorption cross-section σ can be estimated to a first approximation from the saturation behavior of Fig. 2d as . Here, we take for the transmission coefficient at the SiC surface T =0.81. We then fit the experimental data in Fig. 3d using the following set of equations with W S in Equation (3) as the only free parameter: Finally, we fit all the data in Fig. 3c–e allowing to vary σ and a ∞ and using From the best fits, shown by the solid lines in Fig. 3c–e , we obtain W S =75 kW cm −2 and a ∞ =7.5. The obtained value for σ is presented in Table 1 . How to cite this article: Fuchs, F. et al . Engineering near-infrared single-photon emitters with optically active spins in ultrapure silicon carbide. Nat. Commun. 6:7578 doi: 10.1038/ncomms8578 (2015).